Highly stretchable and transparent nanomesh electrodes made by grain boundary lithography Foldable photoelectronics and muscle-like transducers require highly stretchable and transparent electrical conductors. Some conducting oxides are transparent, but not stretchable. Carbon nanotube films, graphene sheets and metal-nanowire meshes can be both stretchable and transparent, but their electrical resistances increase steeply with strain <100%. Here we present highly stretchable and transparent Au nanomesh electrodes on elastomers made by grain boundary lithography. The change in sheet resistance of Au nanomeshes is modest with a one-time strain of ~160% (from ~21 Ω per square to ~67 Ω per square), or after 1,000 cycles at a strain of 50%. The good stretchability lies in two aspects: the stretched nanomesh undergoes instability and deflects out-of-plane, while the substrate stabilizes the rupture of Au wires, forming distributed slits. Larger ratio of mesh-size to wire-width also leads to better stretchability. The highly stretchable and transparent Au nanomesh electrodes are promising for applications in foldable photoelectronics and muscle-like transducers. The development of foldable photoelectronics [1] and muscle-like transducers [2] , [3] , [4] has highlighted a fundamental fact: few electronic conductors are both stretchable and transparent. The existing stretchable and transparent electrodes, such as graphene sheets, carbon nanotube films and metal nanowire networks, suffer from either high sheet resistance or low stretchability [5] , [6] , [7] , [8] , [9] , [10] , [11] , [12] , [13] . The latest understanding is that fully interconnected metal nanowire networks can have good electrical conductance since they do not have the problem of high wire-to-wire junction resistance [13] , [14] , [15] , [16] . While the networks demonstrate good transparency and electrical conductance, their flexibility becomes a more interesting topic. Although metal interconnects are more conductive than the random metal nanowire-networks, it is still a challenge for a metal interconnect to work under ultralarge strains (for example, 100%). Moreover, few reports have offered physical insight for the flexibility of transparent metal interconnects. Therefore, clarifying the underlying physics of the ultrahigh stretchability is of great both scientific and practical importance. Here we present a method called grain boundary lithography, for making metal nanomesh electrodes. The nanomesh is a network of fully interconnected metal wires of gold (Au); it avoids the problem of high junction resistance and has good electrical conductivity as well as transparency. The Au nanomesh exhibits ultrahigh stretchability: it has a modest increase in electrical resistance even if it is stretched to a strain as large as ~160% or after 1,000 cycles at a strain of 50%. The good stretchability results from two facts: the stretched nanomesh adherent on an elastomeric structure undergoes distributed rupture of nanowires and the serpentine nanowires deflect out of the plane. Besides, the Au nanomeshes do not have oxidation problem like Ag and Cu, causing a remarkable decrease of electrical conductivity for Ag and Cu nanowire-networks under a mild temperature of 200 °C or even at room temperature [8] , [16] , [17] . Grain boundary lithography for metal nanomeshes The grain boundary lithography involves a bilayer lift-off metallization process, which offers advantages in resolution, removal, process simplicity, undercut control and yield over conventional single-layer lift-off process [18] , [19] . In this work, the bilayer consists of an In 2 O 3 mask layer and a SiO x sacrificial layer for undercut formation. The In 2 O 3 mask layer is transformed from an In film by HNO 3 etching and thermal oxidation. The as-deposited In film is made of monolayered In grains, and after HNO 3 etching a gap is formed with a controllable width between neighboring grains. 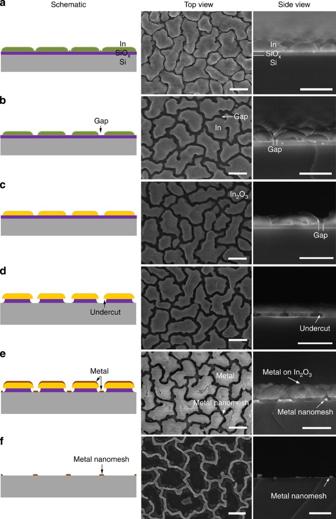Figure 1: Fabrication of metal nanomeshes. The left column represents schematics, while the middle and right columns are corresponding top view and cross-sectional scanning electron microscopy (SEM) images. (a) Deposition of In/SiOxbilayer on a Si wafer. (b) Gap formation by etching in diluted HNO3. (c) Conversion of In islands into In2O3islands by thermal oxidation. (d) Undercut formation by rinsing in diluted HF. (e) Deposition of metal film leading to the formation of metal nanomesh in the grooves. (f) Lift-off process to remove In2O3and SiOx. Scale bar, 500 nm. Figure 1a–f shows the six steps of the grain boundary lithography: (1) deposition of a 65 nm thick SiO x sacrificial layer on Si wafer (resistivity: 5–7 Ω·cm, thickness: 0.5 mm), followed by depositing a 100 nm thick In film; (2) etching in 20 wt.% HNO 3 for gap formation; (3) thermal oxidation at 400 °C for 2 h to form In 2 O 3 islands; (4) rinsing in 5 wt.% HF for 12 s, leading to the formation of undercuts; (5) deposition of metal film of Au on top of the In 2 O 3 film, so that a metal nanomesh is formed in the gaps; and (6) lift-off process to dissolve the SiO x and removal of In 2 O 3 islands in 5% HF solution to form a metal nanomesh on the substrate. Figure 1: Fabrication of metal nanomeshes. The left column represents schematics, while the middle and right columns are corresponding top view and cross-sectional scanning electron microscopy (SEM) images. ( a ) Deposition of In/SiO x bilayer on a Si wafer. ( b ) Gap formation by etching in diluted HNO 3 . ( c ) Conversion of In islands into In 2 O 3 islands by thermal oxidation. ( d ) Undercut formation by rinsing in diluted HF. ( e ) Deposition of metal film leading to the formation of metal nanomesh in the grooves. ( f ) Lift-off process to remove In 2 O 3 and SiO x . Scale bar, 500 nm. Full size image The line width (W), average mesh size (M) and thickness of the metal nanomeshes are all well controlled ( Supplementary Fig. 1 ). The width of the metal wires is defined by the gap in step (2). Our experimental data reveal that the gap width increases linearly with the increase of HNO 3 etching time ( Supplementary Fig. 1d ). The good uniformity and controllability of gap width is related to the isotropic etching process, including surface oxidation (or passivation) and acidic etching ( Supplementary Fig. 1a–c ), expressed as If the etching process does not involve oxidation, then metallic In will be directly etched by H + . Owing to the fact that etching rates differ for different facets, the gap width will therefore not be homogeneous. Moreover, this process will be very fast. For example, 4 mol l −1 HCl solution (a non-oxidizing acid with H + concentration close to that of the HNO 3 solution we used) could dissolve the In film in just 1 s. Alternatively, an oxide skin could lead to isotropic etching that is similar to the isotropic etching of single crystalline Si wafer in HNA solution (blended solution of HF, HNO 3 , and CH 3 COOH, in which HNO 3 is the oxidant) [20] . The surface oxide decreases the etching rate to a controllable level. Moreover, the etching process of a wafer scale sample can be finished in seconds, indicating that this process is quite suitable for mass production. Note that the oxide skin is dynamically formed so that there is always an oxide layer on the In islands. The isotropic etching from grain boundaries offers a much more precise controllability over the width of metal nanowires, and the mechanism is much different from main-stream nanofabrication techniques, for which the feature size is often determined by the spot size of energy beam or by template feature size. The mesh size, which equals to the size of In islands, is found to have a linear relationship with the thickness of the In films, with an empirical relationship of M=7 h , where h is the film thickness is in the range of 50–500 nm. The thickness of the metal nanomeshes can be precisely controlled by varying the metal film thickness. The line width, mesh size and thickness of the metal nanomeshes determine transmittance and sheet resistance. It should be noted that besides indium, other materials with different morphology may also be used as the precursor of the mask layer. This may allow for the fabrication of metal nanomeshes with different topologies, which will affect the electrical conductivity and flexibility of the nanomeshes. Metal nanomesh transfer by wedging transfer To completely remove the In 2 O 3 grains and protect the metal mesh, we use catalytic etching [21] in which the metal nanomesh is buried into Si wafer with a depth of several hundred nanometres. Metal nanomeshes on or embedded inside silicon wafer, however, are difficult to be directly transferred to other substrates because it is difficult to get the nanomesh free. To solve this problem, we first introduce a dissolvable layer (K 2 SiO 3 ) between the metal mesh and Si substrate by chemical reaction of the sample with hot diluted KOH solution (wt. 2%) and then slowly wedge the sample into diluted HF solution (wt. 1%) with an entrance angle of ~30° ( Fig. 2a ) [22] . As the K 2 SiO 3 layer dissolves in HF, the metal nanomesh detaches from the hydrophobic Si surface and floats on the solution ( Fig. 2b ). The metal nanomeshes do not sink in water, and they float on water without folding or wrinkling. This is because water could not penetrate Au nanomeshes, although Au is hydrophilic, as surface tension of water can support the meshes. Moreover, a component of surface tension of water pulls normally and horizontally to each nanowire; and, at a macro level, this force is outwards and perpendicular to the edges of a nanomesh and therefore keeps the nanomesh unfolded. The floating metal nanomesh can then be transferred onto a poly(dimethylsiloxane) (PDMS) layer ( Fig. 2c,d ). 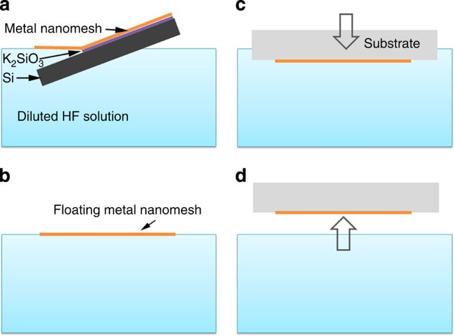Figure 2: Transfer of the metal nanomesh. (a) Wedging transfer of metal nanomesh. (b) Floating metal nanomesh. (c) Pressing a target substrate on the metal nanomesh. (d) Lifting the nanomesh. Figure 2: Transfer of the metal nanomesh. ( a ) Wedging transfer of metal nanomesh. ( b ) Floating metal nanomesh. ( c ) Pressing a target substrate on the metal nanomesh. ( d ) Lifting the nanomesh. Full size image Directly lifting the floating metal mesh with a target substrate from the water side will introduce a water membrane between metal nanomesh and the substrate, and this might further lead to the formation of wrinkles or folds during drying (graphene flakes transferred by this method often have wrinkles) [22] , [23] , or even rupture. To avoid damage or deformation, the substrate should not contact water. We use the substrate to contact the metal nanomesh from the air side ( Fig. 2c,d ). Our experimental results show that this simple method is effective and capable of transferring metal nanomeshes onto hydrophobic (PDMS) or hydrophilic (metal) substrate without damage or deformation. We can also directly cast uncured PDMS on the Au nanomesh/K 2 SiO 3 /Si wafer. After curing of PDMS, the K 2 SiO 3 layer can then be dissolved and Au/PDMS can be detached. However, in this case, the PDMS surface is not very flat and thus the transmittance is not good. Super-flexibility of Au nanomeshes The nanomeshes of Au have excellent electrical conductivity. For a 50-nm thick Au nanomesh with a mesh size of ~700 nm and a line-width of ~90 nm, the lowest sheet resistance ever obtained is ~7 Ω per square (sq). This is lower than that of carbon nanotube- and graphene-based transparent electrodes (>100 Ω per sq) [24] , commercial ITO films (15–50 Ω per sq) and solution-processed Au nanomeshes (>400 Ω per sq) [25] , and comparable to Ag nanonetworks with similar features made by electron beam lithography, which do not have contact junction problem [26] . The low resistance should be related to the absence of high junction resistance between the wires. The electrical conductivity of the nanomeshes can be further tuned to a higher level by making the nanomesh line width larger and/or film thicker. Au has excellent ductility and hence was used for ultra-thin foils in ancient times, and a recent work has confirmed the superplasticity of Au nanowires [27] . 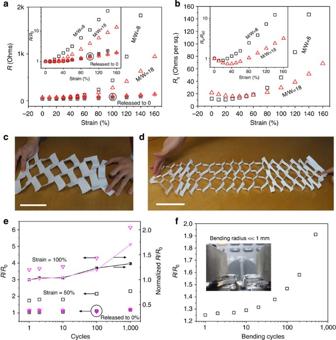Figure 3: Flexibility and resistance of nanomeshes. (a)RandR/R0(inset) as a function of tensile strain. The Au nanomesh with a mesh-size to line-width ratio (M/W) of 18 (red triangles) has aR/R0of only 13.3 as the sample is stretched to a strain of 160%. Another Au nanomesh sample with a lower M/W of 8 (black squares) presents worse stretchability. (b)RsandRs/Rs0(inset) as a function of tensile strain for Au nanomeshes. The sample with an M/W ratio of 18 shows aRs/Rs0of only 3.2 when it is stretched to 160%; andRsis even lower thanRs0below 80% strain. The sample with M/W of 8 reveals a higher sheet resistance change, which reaches 12.3 at a strain of 140%. (c) and (d) Stretching two sheets of letter-sized papers containing an array of slits with coarse and fine ligaments, respectively. The closely spaced slits appear to be much more stretchable. Scale bar, 10 cm. (e) Change in resistance versus cycles (up to 1,000 cycles) of two Au nanomesh samples with M/W of 18, normalizedR/R0is also shown. Magenta symbols represent 100% strain while black symbols represent 50% strain. (f)R/R0as a function of bending cycles. The sample is bent to a ‘V’ shape (inset) so that the bending radius is far smaller than 1 mm (the Au nanomesh is on the top side). After 500 cycles of bending,R/R0has an acceptable increase to 1.9. Figure 3a plots the dependence of resistance ( R ) on tensile strain ( ɛ ) for Au nanomeshes of ~7 mm long and ~2 mm wide on ~1 mm thick PDMS substrate ( R 0 is the initial resistance of ~70 Ω for sample with W/M=18 and ~40 Ω for W/M=8, here M/W is the ratio of mesh-size to line-width). The ratio of R / R 0 of the Au nanomesh with M/W of 18 is only ~3.8 at a strain of 100%, and it increases to 13.3 at an ultra-large strain of 160%, as shown in the inset of Fig. 3a . This is better than the Ag nanomesh made of ‘very long Ag nanowires’, for which resistance sharply increases ( R / R 0 >100) as stretched by 90% (ref. 28 ). There are only a few existing transparent conductors that can work at a strain of 100%, such as a graphene-metal nanowire hybrid structure [29] . It is worth pointing out that the increased resistance almost disappears when the strain is fully released, shown by the ‘+’ centred symbols, probably because of the re-contact and cold welding of fractured nanowire where necking happened. This is evidenced by the fact that it takes time for R (after releasing the stress) to get stabilized. Au could not be oxidized in air so that no oxide skin will be formed, and this makes cold welding possible. Supplementary Fig. 2 shows that released Au nanomesh has morphology quite similar to non-stretched sample, without large cracks, indicating re-contact and cold welding. The details of the microstructure of nanowire necking and fracturing under large strain, and cold welding upon strain release will be published separately. The low ratio of R / R 0 (after strain release) is very important because it means that Au nanomesh can recover from damage. Figure 3: Flexibility and resistance of nanomeshes. ( a ) R and R / R 0 (inset) as a function of tensile strain. The Au nanomesh with a mesh-size to line-width ratio (M/W) of 18 (red triangles) has a R / R 0 of only 13.3 as the sample is stretched to a strain of 160%. Another Au nanomesh sample with a lower M/W of 8 (black squares) presents worse stretchability. ( b ) R s and R s / R s0 (inset) as a function of tensile strain for Au nanomeshes. The sample with an M/W ratio of 18 shows a R s / R s0 of only 3.2 when it is stretched to 160%; and R s is even lower than R s0 below 80% strain. The sample with M/W of 8 reveals a higher sheet resistance change, which reaches 12.3 at a strain of 140%. ( c ) and ( d ) Stretching two sheets of letter-sized papers containing an array of slits with coarse and fine ligaments, respectively. The closely spaced slits appear to be much more stretchable. Scale bar, 10 cm. ( e ) Change in resistance versus cycles (up to 1,000 cycles) of two Au nanomesh samples with M/W of 18, normalized R / R 0 is also shown. Magenta symbols represent 100% strain while black symbols represent 50% strain. ( f ) R / R 0 as a function of bending cycles. The sample is bent to a ‘V’ shape (inset) so that the bending radius is far smaller than 1 mm (the Au nanomesh is on the top side). After 500 cycles of bending, R / R 0 has an acceptable increase to 1.9. Full size image The sheet resistance ( R s ) of the stretched Au nanomesh is even smaller than the original sheet resistance ( R s0 =21 Ω per sq for W/M=18) until it is stretched to 80% ( Fig. 3b ). This means that the Au nanomesh is even ‘more conductive’ when stretched to relatively low strains. From Fig. 3a , it is easy to understand the decrease in R s / R s0 because the resistance R does not change too much, but the dimensions change a lot when the strain reaches 40% at which the Au nanowires are only straightened or reoriented to comply with the stretching without significant plastic elongation or fracture. Beyond 40%, the Au nanowires undergo damage so that the resistance increases much faster ( Fig. 3a ), and the increase in sheet resistance over-rides the effect of dimensional deformation at ~80%. We can see that the ratio of R s / R s0 is only 3.2 as strain goes to 160%, much smaller than 13.3 of R / R 0 . We also find that M/W could significantly affect the flexibility of the Au nanomeshes. Figure 3a,b shows data of two Au nanomeshes with M/W of 18 and 8. At large strains, the sample with larger M/W presents much smaller R / R 0 and R s / R s0 values. This observation can be understood by a simple demonstration: the sheet of paper cut with more closely spaced slits (larger M/W, Fig. 3d ) is more stretchable than the sparsely cut one ( Fig. 3c ). Au nanomeshes also perform well under cyclic strain ( Fig. 3e ). The sample does not experience obvious fatigue at 50% tensile strain. In comparison, R / R 0 significantly changes at 100% strain after 1,000 cycles. However, change of the resistance after releasing load is modest, even for the sample stretched at 100% strain for 1,000 cycles ( R / R 0 slightly changes from 1.15 to 1.21). We also performed cyclic bending experiments. A Au nanomesh bent to ‘V’ shape with a bending radius far smaller than 1 mm only has a R / R 0 of 1.9 after 500 cycles of bending ( Fig. 3f ). Keeping good electrical conductivity with bending radius on submillimeter scale is highly desired in foldable electronics. Transmittance of Au nanomeshes The Au nanomesh also presents a high specular transmittance of 82.5% (at a sheet resistance of ~20 Ω per sq) in the wavelength range of 400–1,000 nm ( Fig. 4 ), which does not include scattered transmission portion. For Ag nanomeshes made of solution processed nanowires, scattered transmission is often more than 10% (ref. 12 ). Even when the total transmittance achieves 90%, the specular transmission is ~80%. In comparison, scattered transmission for our Au nanomesh is only ~3% for the portion scattered out of the solid angle ~0.2 steradian (when transmittance exceeds 80%, see Supplementary Fig. 3 ), this may allow its applications in displays or other fields where scattered light is undesired. In addition, we have found that the stretched Au nanomesh has a higher transmittance (from 82.5 to 85.0%) when stretched to ~80% strain. Note that within a strain of 80%, both sheet resistance and transmittance are improved. The higher transmittance of Au nanomesh is related to its low reflectance, which is 5.5% in the range of 400–1,000 nm, measured by an integrating sphere. 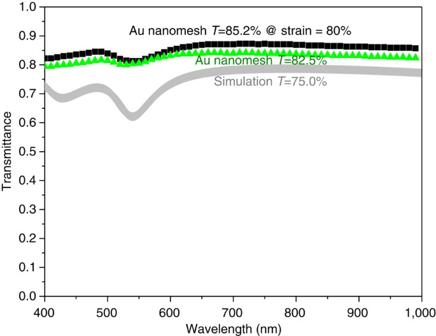Figure 4: Transmittance spectra. In the wavelength range of 400–1,000 nm, the Au nanomesh presents a transmittance of 82.5% (green triangles), close to the simulated result (~75.0%) (grey line). The transmittance of the Au nanomesh becomes larger after stretching (it changes from 82.5 to 85.0% (dark line) with strain changes from 0 to 80%). Figure 4: Transmittance spectra. In the wavelength range of 400–1,000 nm, the Au nanomesh presents a transmittance of 82.5% (green triangles), close to the simulated result (~75.0%) (grey line). The transmittance of the Au nanomesh becomes larger after stretching (it changes from 82.5 to 85.0% (dark line) with strain changes from 0 to 80%). Full size image Mechanism of the super-flexibility of Au nanomeshes The large stretchability of the Au mesh on the PDMS substrate results from two aspects of the structure. First, the Au mesh is a two-dimensional network of curved wires of a metal. When stretch is small, the mesh deforms within the plane. When stretch is large, however, the planar deformation is unstable, and the wires bend and twist out of the plane [30] . It is this out-of-plane deformation that enables the mesh to stretch greatly, as illustrated by a sheet of paper cut with an array of slits ( Fig. 3c or d ). The larger the mesh size-to-width ratio (W/M), the more stretchable is the sheet. Second, the Au mesh is adherent to the PDMS substrate. Because the elastic modulus of Au is about five orders of magnitude larger than that of PDMS, the substrate readily accommodates the out-of-plane deflection of the mesh [30] . The PDMS substrate, however, serves a significant function: it creates distributed rupture of Au ligaments. To illustrate this function, we cut a sheet of paper with a laser mimicking a magnified image of the Au mesh ( Fig. 5a ). The size of the paper ligaments is about ten thousand times the Au wires. The paper mesh can only be stretched to about 20% and then breaks into two halves. Once we use scissors to cut some ligaments, the mesh behaves in a similar way as the sheet containing long, closely-spaced slits and becomes much more stretchable. This demonstration illustrates a principle: if the mesh could break ligaments here and there gradually, it would be stretched greatly. In a freestanding mesh, however, once a long slit forms, the stress concentrates in the ligament at a tip of the slit, so that this ligament will break, and the localized damage will break the mesh into two halves. By contrast, for a mesh on a soft substrate, the substrate stabilizes any large slit and allows ligaments elsewhere to rupture. This phenomenon is reminiscent of the rupture in a metal film on a polymer substrate [31] , [32] , or that in highly stretchable hydrogels [33] , [34] . This mechanism ensures that the Au nanomesh on PDMS will still be conductive even stretched to strains beyond 160%. 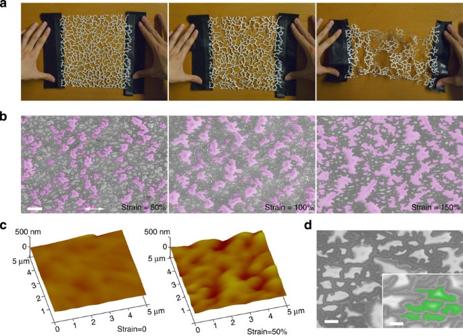Figure 5: Distributed rupture and formation of nested self-similar mesh. (a) A sheet of paper is laser-cut using the magnified image of Au nanomesh. The left image shows without any cutting. The middle image shows the stretching of the structure after cutting a few ligaments. The right image shows the stretching of the structure after cutting more ligaments. (b) Au nanomesh/PDMS stretched at strains of 50, 100 and 150%, showing that cracks (filled with purple) are formed and the crack size increases with increasing strain. The double headed arrow indicates tensile direction. Under large strains of 100 and 150%, a larger mesh is formed, for which the cracks act as the holes (purple) while the non-cracked Au networks and wires act as larger ligaments (dark grey). Scale bar, 3 μm. (c) Atomic force microscopy images of unstretched and stretched Au nanomesh supported on PDMS, showing that the latter has a relief height up to 200 nm. (d) Straight nanowires and elongated meshes (exemplified by the mesh in green in the inset) are seen in strained Au nanomesh (at a strain of 150%). Scale bar, 1 μm, and scale bar in the inset is 500 nm. Figure 5: Distributed rupture and formation of nested self-similar mesh. ( a ) A sheet of paper is laser-cut using the magnified image of Au nanomesh. The left image shows without any cutting. The middle image shows the stretching of the structure after cutting a few ligaments. The right image shows the stretching of the structure after cutting more ligaments. ( b ) Au nanomesh/PDMS stretched at strains of 50, 100 and 150%, showing that cracks (filled with purple) are formed and the crack size increases with increasing strain. The double headed arrow indicates tensile direction. Under large strains of 100 and 150%, a larger mesh is formed, for which the cracks act as the holes (purple) while the non-cracked Au networks and wires act as larger ligaments (dark grey). Scale bar, 3 μm. ( c ) Atomic force microscopy images of unstretched and stretched Au nanomesh supported on PDMS, showing that the latter has a relief height up to 200 nm. ( d ) Straight nanowires and elongated meshes (exemplified by the mesh in green in the inset) are seen in strained Au nanomesh (at a strain of 150%). Scale bar, 1 μm, and scale bar in the inset is 500 nm. Full size image Our experimental results with nanomeshes support the distributed rupture and out-of-plane mechanism, which is supported by the observation of the evolution of distributed pockets using SEM ( Fig. 5b ), and that of the out-of-plane deformation using atomic force microscope (AFM) ( Fig. 5c ). The magnitude of out-of-plane deformation is on the order of the ligament width as is predicted in theoretical calculations [30] . The resistance goes up steadily at large strain ( Fig. 3a,b ). At small strain, the stretch of each ligament and the deformation of each mesh pore can also contribute to the stretchability, so that only at large strain does our distributed rupture mechanism shows dominating effect. Elongation of the mesh pores still contribute to the stretchability at large strain ( Fig. 5d ). Such a mechanism can also explain the cyclic behaviour we observed. After breaking a few ligaments and forming the slits, the deformation of the thin film is elastic, as is demonstrated by our paper samples. In addition, based on our paper model ( Fig. 3c,d ), we can roughly estimate that the radius of curvature of the thin film should scale with the mesh size. Since our film thickness is much smaller than the mesh size, the strain in the gold film should be generally small. As a result, there is almost no fatigue effect even for cyclic strain as large as 50% ( Fig. 3e ). However, due to the random nature of our meshed structures and touch of some nanowires, we do expect stress concentration on some sites. Over cycles, these high strain sites could fail due to fatigue. As discussed above, these failure sites are delocalized due to the presence of the substrate. Evidently, the higher the overall strain, the more sites are likely to be under high strain. This explains why for 100% strain the fatigue effect is much significant. The two aspects of the structure—out-of-plane deformation and delocalized rupture—are insensitive to geometric details of the mesh. The geometric details of the mesh, however, may affect the stretch-resistance behaviour quantitatively. In particular, it will be instructive to study the effect of bimodal or multimodal distribution of sizes and of multiscale irregularities. It is interesting that under large strains of 100 and 150% a larger mesh is formed (because the substrate delocalizes the rupture of Au nanomesh), for which the cracks act as the holes while the non-cracked Au networks act as larger ligaments ( Fig. 5b ). The larger mesh is quite similar to the original nanomesh and this allows the electrode behaving like the case at small strains, and therefore it can be further stretched to larger strains while being electrically conductive before failure of the substrate. It is worth noting that adhesion between Au nanomesh and the PDMS substrate plays an important role. The right adhesion creates distributed rupture of the nanomesh and thereby leads to high stretchability; either too weak or too strong adhesion decreases the flexibility significantly. Surface modification of PDMS could change the adhesion and hence tune the stretchability, and the quantitative effect of adhesion on flexibility is being studied and will be reported in details in the future. In addition, surface pattern may help to get a better stretchability. However, compared with the distributed rupture mechanism, the enhancement is limited. While adding the surface roughness will cause some adhesion problems, which may compromise the benefits of rough surfaces. High thermal stability The Au nanomesh also presents good thermal stability. Metals of Ag and Cu nanomeshes are prone to oxidation leading to deterioration of electrical and optical properties. For example, solution processed Ag nanomeshes have a marked decrease in conductivity when annealed at 200 °C or higher for more than 20 min (ref. 16 ). Cu nanowires are severely oxidized even at room temperature within days without protection [8] , [17] . In comparison, Au nanomeshes do not have this oxidation problem and can work at temperatures up to 500 °C ( Supplementary Fig. 4 ), and their electrical conductivity can even be improved with thermal annealing. Although Au is more expensive, the price is affordable when the nanomesh is thin, and the material actually contributes only a small portion of the total cost in thin film technology. In addition, compared with metal nanomeshes made of solution processed metal nanowires, which are quite rough, our metal nanomeshes are more compatible to lithographic process and are possibly used to make microcircuit with a feature size of several microns, which is unavailable by using solution processed Ag nanowire networks. In conclusion, we have introduced grain boundary lithography to fabricate Au nanomesh electrodes with excellent mechanical stretchability, electrical conductivity and optical transparency. Through macroscopic observations of laser-cut paper and microscopic observations of nanomeshes, we find that the large stretchability of Au nanomeshes results from a subtle balance of two roles played by the PDMS substrate. The vast difference in the elastic moduli of Au and PDMS allows the stretched Au mesh to deflect out of the plane, while the substrate stabilizes distributed rupture of Au ligaments. A nested self-similar mesh is formed at quite large strains and this allows the electrode behaving like the case at small strains, and therefore it can be further stretched to larger strains. This work shows that the Au nanomesh electrodes are promising for applications in foldable photoelectronics and muscle-like transducers. Fabrication and transfer of floating Au nanomeshes The SiO x film (65 nm) and In film (~100 nm) were deposited by using a magnetron sputter (AJA International, ORION-8 magnetron sputtering system), and the Au films were deposited by using an electron beam evaporation system (Edwards BOC-500). The floating metal nanomeshes were made by following three steps: (1) rinsing the samples in blended solution of HF (10%) and H 2 O 2 (0.6%) for 2 min, (2) rinsing in 60 °C KOH (2%) solution until the sample turned from black to grey and drying with N 2 gas flow, (3) wedging into diluted HF (1%) slowly. The metal nanomesh was then transferred to hydrophobic or hydrophilic substrate by slowly pressing the substrate on the floated nanomesh and lifted after it was attached to the substrate. Characterization Morphology of the samples was recorded by using a JEOL 6340F and a Hitachi S-4800 scanning electron microscope. Topographic images were taken with a Veeco D-3100 atomic force microscope. Sheet resistance was measured by using the van der Pauw method, with four electrodes at four corners of a square of the sample and recorded with a Keithley 2400, meter and an Agilent 34401A meter. Optical spectra were recorded with an integrating sphere spectrometer (Ocean Optics, USB4000 VIS-NIR-ES, ISP-REF) in the wavelength range from 400 to 1,000 nm. After wedging transfer, the Au/PDMS was cut into strips, typically with a length of 5–10 mm, width of 1–3 mm and thickness of 0.5–1 mm for property tests under deformation. Stretching and bending experiments were conducted with a home-made setup, and meanwhile the resistance was measured by a two-probe method. Optical simulation The simulation for the optical transmittance of the gold nanomeshes was performed on Computer Simulation Technology (CST) Microwave Studio, a finite difference time domain and finite difference frequency domain software. To perform the simulation, we traced the edges of a Au nanomesh (about 8.5 μm × 2.7 μm), and sections of the polygon are used as unit cells to be simulated. Figure 4 was obtained from average of multiple simulations. How to cite this article: Guo, C. F. et al. Highly stretchable and transparent nanomesh electrodes made by grain boundary lithography. Nat. Commun. 5:3121 doi: 10.1038/ncomms4121 (2014).